PD-L1hiB cells are critical regulators of humoral immunity Specific B-cell subsets can regulate T-cell immune responses, and are termed regulatory B cells (Breg). The majority of Breg cells described in mouse and man have been identified by IL-10 production and are known to suppress allergy and autoimmunity. However, Breg cell mediated immune suppression, independent of IL-10, also occurs. Here we show that Breg cells play a critical role in regulating humoral immunity mediated by CD4 + CXCR5 + PD-1 + follicular helper T cells, and can suppress inflammation in autoimmune disease through elevated expression of PD-L1. We have also identified that these B cells are resistant to αCD20 B-cell depletion. This work describes how Breg cells are critical in humoral homoeostasis and may have implications for the regulation of autoimmune diseases. Classically, B cells are considered to be potent antibody producers. However, specific B-cell subsets can also negatively regulate T-cell immune responses, and have been termed regulatory B cells (Breg) [1] , [2] , [3] . A part of the humoral immune response is the interaction between follicular helper T cells (T FH cells) and cognate B cells to drive the formation and maintenance of germinal centre (GC) reactions [4] , [5] , [6] , [7] . T FH cells express the chemokine receptor CXCR5, which directs them to B-cell follicles via gradients of the chemokine CXCL13 (refs 4 , 5 ). T FH cells also express the transcription factor Bcl-6 and have high expression of the co-stimulatory receptor ICOS. Both Bcl-6 and ICOS [8] , [9] , and more recently Ascl2 (ref. 10 ) have been described as being critical for the differentiation and maintenance of T FH cells. In humans and mice, functionally similar T FH cells can be found in secondary lymphoid organs. In several autoimmune conditions the levels of circulating CXCR5 + T FH cells are elevated and T FH cells have been correlated to antibody responses in HIV [11] , [12] . Another characteristic feature of T FH cells is their elevated expression of the inhibitory receptor programmed death receptor-1 (PD-1). PD-1 has two ligands, PD-L1 (B7-H1) and PD-L2 (B7-DC), which are expressed to varying degrees across epithelial and haematopoietic cell populations [13] . Signalling through PD-1 is known to attenuate signalling from the T-cell antigen receptor (TCR) and inhibits the population expansion, cytokine production and cytolytic function of T cells [14] . Studies of PD-1 receptor: ligand interactions have suggested the importance of this pathway in regulating humoral immune responses. Previously, we and others, have shown that PD-L1 regulates T FH -cell expansion and subsequent antibody responses to both model [15] and helminth-derived antigens [16] . More recently PD-1/PD-L1 interactions have been identified as having roles in the generation of a CD4 + CXCR5 + subset of cells called ‘follicular regulatory T cells’ (T FR cells), which express the transcription factors Foxp3, Bcl-6 and Blimp1 and function to inhibit the GC response [17] , [18] . These recent findings have demonstrated the importance of T-cell subsets regulating the GC and humoral response. However, there has been little focus on Breg cell populations and their respective ability to regulate T FH -cell expansion and subsequent antibody responses. Here we are able to describe the importance of PD-L1 expression on B cells in the context of humoral immunity and autoimmune disease in both mouse and man. Our studies demonstrate that elevated PD-L1 expression on B cells is an important regulator of T FH -cell activity, downstream antibody responses and subsequent disease progression. Through the use of transfer approaches it is demonstrated that Breg cells which express high levels of PD-L1 (PD-L1 hi ), dramatically suppress humoral responses through attenuating the activation of T cells and antibody production, independent of other reported suppressor populations [17] , [18] , [19] . Using an experimental model of autoimmune disease we demonstrate that PD-L1 hi Breg cells can suppress the incidence and severity of disease. We further found that PD-L1 hi Breg cells were refractory to B-cell depletion therapy (αCD20 monoclonal antibody (mAb) treatment). The suppressive capacity of these Breg cells was demonstrated to be dependent on PD-L1. The retention of PD-L1 hi Breg cells, post B-cell depletion therapy, was attributed to elevated expression of the B-cell activating factor (BAFF) receptors BAFF-R, TACI and BCMA, which displayed enhanced uptake of BAFF compared with other B-cell subsets. Together, our studies identify that Breg cells can suppress through the PD-1/PD-L1 pathway in limiting the differentiation and function of T FH cells. It also demonstrates a novel mechanism by which B-cell depletion therapy works, and thus provides insight into the dynamic control of humoral immune responses in both homoeostasis and disease. B-cell PD-L1 expression regulates humoral immunity T FH cells, and by extension the propensity to develop a humoral immune response, require several different signals to proliferate and provide adequate B-cell help [6] , [20] . PD-L1 has previously been reported to regulate T FH expansion [15] , [16] . As PD-L1 can be expressed by many types of haematopoietic cells, including T cells, B cells, macrophages and some dendritic cells [13] , we investigated whether B-cell-specific PD-L1 regulates T FH cells directly by controlling their expansion. To demonstrate the effect of PD-L1 expression on B cells in humoral immunity, mixed-bone marrow chimeric mice were generated ( Supplementary Fig. 1a ) with a B-cell-specific deficiency in PD-L1 (B-PD-L1 −/− ) and control chimeras (B-wild type (B-WT)). After 10 weeks of reconstitution (confirmed via flow cytometry; Supplementary Fig. 1b ), chimeric mice were immunized with keyhole-limpet haemocyanin emulsified in complete Freund’s adjuvant (KLH/CFA), an immunization which is known to evoke generation of T FH cells after 14 days [16] . T FH cells were defined as CD4 + B220 − CXCR5 + PD-1 + ( Supplementary Fig. 1c ). Consistent with previous reports, T FH cells expressed high levels of ICOS, possess the transcription factor Bcl-6 and produce IL-21. Immunization with KLH/CFA led to a significant increase in both the proportion and number of T FH cells in both the spleen ( Supplementary Fig. 1d,e ) and the draining lymph node (dLN) ( Supplementary Fig. 1f,g ) in B-PD-L1 −/− mice relative to B-WT mice. To assess whether the marked expansion of T FH cells in immunized B-PD-L1 −/− influenced the magnitude of the immunoglobulin (Ig) response, we measured KLH-specific IgG, IgG1 and IgG2a. B-PD-L1 −/− had significantly elevated antigen-specific Ig production compared with comparable immunized B-WT ( Supplementary Fig. 1h–j ). Comparisons between immunized Pdl1 −/− and B-PD-L1 −/− animals demonstrated a significant role for PD-L1 expression on B cells with both groups exhibiting expansion in T FH cells following immunization, as demonstrated previously [16] ( Supplementary Fig. 2a–h ). This supports the notion that PD-L1 expressed on B cells has a role in regulating T FH -cell expansion and downstream Ig production. PD-L1 is differentially expressed on B cells The expression of PD-L1 compartmentalizes B cells into three distinct (PD-L1 lo , PD-L1 int and PD-L1 hi ) populations ( Fig. 1a ). Using flow cytometry, PD-L1 hi B cells were cell surface phenotyped based on known B-cell subsets: transitional 1/2; marginal zone (MZ); follicular origin; B1/B2 and GC cells ( Fig. 1b ). PD-L1 hi expressing B cells are found within the MZ (CD19 + CD23 + CD21 +/hi IgM +/hi ) and MZ-progenitor (CD19 + CD23 − CD21 + IgM + ) compartments, similar to other described Breg cells [21] , [22] , [23] . PD-L1 hi B cells are also B2-B cells (CD19 + IgM + CD5 − CD11b − ) with a small population (0.3%±0.2) detected as GC B cells (CD19 + CD95 + GL-7 + ). PD-L1 is known to be highly expressed on antibody-secreting cells (ASC), with critical interactions required with T FH cells [15] , [24] and even demonstrating immune suppressive properties in the gut [25] . To formally demonstrate whether CD19 + PD-L1 hi B cells were ASC (Blimp1 + , CD138 + , B220 lo ), Blimp1–enhanced yellow fluorescent protein (Blimp1–eYFP) transgenic mice, previously used to track ASC generation and trafficking [26] , [27] , were immunized with KLH/CFA for 14 days. CD19 + PD-L1 hi B cells isolated after immunization expressed low levels of Blimp1 and CD138 but high levels of B220 ( Fig. 1c ). Furthermore, Blimp1 expressing CD19 + PD-L1 hi cells were isolated and their lymphocyte-like morphology was distinct from the enlarged perinuclear cytoplasm characteristics of Blimp1 + CD138 + B220 lo ASC ( Fig. 1d,e ). 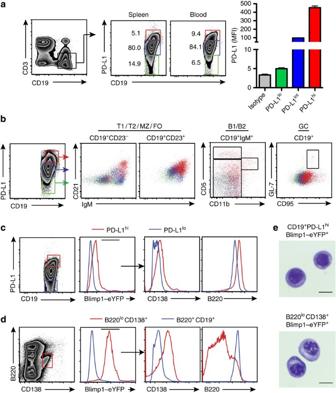Figure 1: B cells express differential amounts of PD-L1. (a) PD-L1 expression on CD3−CD19+cells from the spleen of naïve, C57BL/6 mice yields three distinct populations (PD-L1lo, green; PD-L1int, blue; PD-L1hi, red); numbers adjacent to gates define percentage of total CD3−CD19+cells. Graph depicts the median fluorescent intensity of PD-L1 on CD3−CD19+cells. Data is representative of six mice (error bars, s.e.m.) (b) Overlaid flow cytometry plots phenotyping major B-cell subsets. CD19+PD-L1lo/int/hiB cells were gated as CD23+/−before comparison of CD21 and IgM expression. Cells were also phenotyped for B1/B2 (CD11b versus CD5) classification and identification as germinal center B cells (CD95+GL-7+) (PD-L1lo, green; PD-L1int, blue; PD-L1hi, red). (c) PD-L1lo(blue) and PD-L1hiB cells (red) were analyzed via flow cytometry for Blimp1, CD138 and B220 and compared with ASCs (d). (e) Images of Blimp1+CD19+PD-L1hiB cells and Blimp1+B220loCD138+cells from KLH/CFA-immunized Blimp1–eYFP reporter mice stained using the Kwik-Diff cell differentiation kit. Scale bar, 5 μm. Representative plots and images are shown for four mice. Figure 1: B cells express differential amounts of PD-L1. ( a ) PD-L1 expression on CD3 − CD19 + cells from the spleen of naïve, C57BL/6 mice yields three distinct populations (PD-L1 lo , green; PD-L1 int , blue; PD-L1 hi , red); numbers adjacent to gates define percentage of total CD3 − CD19 + cells. Graph depicts the median fluorescent intensity of PD-L1 on CD3 − CD19 + cells. Data is representative of six mice (error bars, s.e.m.) ( b ) Overlaid flow cytometry plots phenotyping major B-cell subsets. CD19 + PD-L1 lo/int/hi B cells were gated as CD23 +/− before comparison of CD21 and IgM expression. Cells were also phenotyped for B1/B2 (CD11b versus CD5) classification and identification as germinal center B cells (CD95 + GL-7 + ) (PD-L1 lo , green; PD-L1 int , blue; PD-L1 hi , red). ( c ) PD-L1 lo (blue) and PD-L1 hi B cells (red) were analyzed via flow cytometry for Blimp1, CD138 and B220 and compared with ASCs ( d ). ( e ) Images of Blimp1 + CD19 + PD-L1 hi B cells and Blimp1 + B220 lo CD138 + cells from KLH/CFA-immunized Blimp1 – eYFP reporter mice stained using the Kwik-Diff cell differentiation kit. Scale bar, 5 μm. Representative plots and images are shown for four mice. Full size image PD-L1 hi B cells exhibited a significantly lower proliferative capacity in response to αIgM/αCD40 stimulation ( Supplementary Fig. 3a ) compared with PD-L1 lo and PD-L1 int subsets. The cytokine profiles of PD-L1-expressing B-cell subsets were also characterized ( Supplementary Fig. 3b ). PD-L1 hi B cells produce significantly more IL-6 and CXCL13 compared with low and intermediate expressing subsets. Interestingly, PD-L1 int B cells expressed significantly more IL-10 than either PD-L1 lo or PD-L1 hi subsets. This suggests that IL-10 may not be a significant mode of suppression for PD-L1 hi B cells. To evaluate whether the IL-10 culture supernatant data was an artifact of the stimuli employed, the proportion of IL-10 competent cells within each PD-L1-expressing subset were determined using IL-10 reporter (10BiT; ref. 28 ) mice. Stimulation of B cells from 10BiT mice revealed that PD-L1 hi B cells contained a smaller proportion of IL-10 competent cells compared with PD-L1 int B cells thus validating the cytokine data described above. Collectively, these data indicate that PD-L1 hi B cells, which constitute 5.2% (±2.3%) of the total splenic CD3 − CD19 + cell population are a MZ B cell, similar to previously reported Breg cells [21] , [22] , [23] . However, these cells demonstrate a lower competence for IL-10 production, suggesting that PD-L1 maybe an alternative suppressive mechanism. Given the propensity of T FH cells to express high levels of PD-1 (ref. 29 ), we sought to demonstrate a role for PD-L1 hi B cells in the regulation of T FH cells and the subsequent downstream humoral immune response. PD-L1 hi B cells regulate T FH -cell expansion To address the functional importance of the differential PD-L1 expression on B cells, adoptive transfer experiments of PD-L1 lo , PD-L1 int and PD-L1 hi B cells in a dose-dependent manner were conducted in KLH/CFA-immunized WT animals. Transfer of PD-L1 hi B cells significantly suppressed KLH-specific Ig production compared with recipients of PD-L1 lo and PD-L1 int B cells, in a dose-dependent manner ( Fig. 2a , Supplementary Fig. 4a ). On analysis of spleen ( Fig. 2b ) and dLN ( Fig. 2c ) T-cell populations, transfer of PD-L1 hi B cells markedly suppressed both the proportion and number of T FH cells and in a dose-dependent manner ( Supplementary Fig. 4a ). 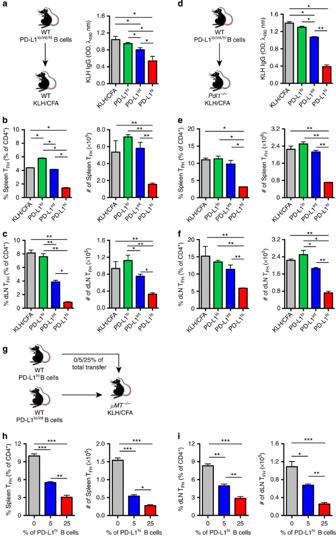Figure 2: High PD-L1-expressing B cells regulate the humoral response. KLH-specific IgG production was evaluated via ELISA following transfer of 1 × 106cells of each PD-L1-expressing B-cell subset into WT KLH/CFA-immunized mice (a). Quantification of TFHcells in the spleen (b) and dLN (c). KLH-specific IgG production was evaluated via ELISA following transfer of 1 × 106PD-L1hiB cells into KLH/CFA-immunizedPdl1−/−animals (d). Quantification of TFHcells from the spleen (e) and dLN (f) immunizedPdl1−/−mice. (g) PD-L1lo/intCD3−CD19+cells were adoptively transferred intoμMT−/−mice. Mice received PD-L1hiB cells as a proportion of total B cells (0, 5 or 25%) followed by immunization with KLH/CFA. TFHcells were quantified in the spleen (h) and dLN (i). *P<0.05, **P<0.01 and ***P<0.001 (Student’st-test). Data are representative of three experiments with six mice per group (error bars, s.e.m.). Figure 2: High PD-L1-expressing B cells regulate the humoral response. KLH-specific IgG production was evaluated via ELISA following transfer of 1 × 10 6 cells of each PD-L1-expressing B-cell subset into WT KLH/CFA-immunized mice ( a ). Quantification of T FH cells in the spleen ( b ) and dLN ( c ). KLH-specific IgG production was evaluated via ELISA following transfer of 1 × 10 6 PD-L1 hi B cells into KLH/CFA-immunized Pdl1 −/− animals ( d ). Quantification of T FH cells from the spleen ( e ) and dLN ( f ) immunized Pdl1 −/− mice. ( g ) PD-L1 lo/int CD3 − CD19 + cells were adoptively transferred into μMT −/− mice. Mice received PD-L1 hi B cells as a proportion of total B cells (0, 5 or 25%) followed by immunization with KLH/CFA. T FH cells were quantified in the spleen ( h ) and dLN ( i ). * P <0.05, ** P <0.01 and *** P <0.001 (Student’s t -test). Data are representative of three experiments with six mice per group (error bars, s.e.m.). Full size image As described above, KLH/CFA-immunized Pdl1 −/− mice demonstrated elevated KLH-specific Ig and increased T FH cells ( Supplementary Fig. 2 ). Adoptive transfer experiments of PD-L1 lo , PD-L1 int and PD-L1 hi B cells into immunized Pdl1 −/− animals demonstrated that PD-L1 hi B cells were able to attenuate, but not completely suppress, Ig production ( Fig. 2d ) and T FH -cell expansion in both the spleen ( Fig. 2e ) and dLN ( Fig. 2f ), whereas transfer of PD-L1 lo and PD-L1 int B cells failed to do so. As transfer of low numbers (1 × 10 5 ) of PD-L1 hi B cells resulted in significant levels of KLH-Ig and T FH suppression ( Supplementary Fig. 4a,b ), we sought to investigate whether adoptive transfer of these cells was providing unprecedented access to sites previously unavailable to native PD-L1 hi B cells. To do this, PD-L1 hi B cells from CD45.1 + transgenic mice were transferred into CD45.2 + animals via either the intravenous or intraperitoneal route to account for cell localization. Immunized subjects were then examined for the location of the transferred cells via CD45.1 + expression ( Supplementary Fig. 2i,j ). CD45.1 + PD-L1 hi B cells were identified in the spleen, dLN and blood, irrespective of the route of administration. This suggests that following transfer, PD-L1 hi B cells disseminate to different tissues where they could contribute to the effects described above. To further confirm PD-L1 hi B cells were suppressive in vivo , a B-cell mixture (total cell number, 1 × 10 7 ) that contained PD-L1 lo/int B cells together with a titration of PD-L1 hi B cells was adoptively transferred into B-cell-deficient (μMT −/− ) mice and immunized with KLH/CFA ( Fig. 2g ). As described above, transfer of PD-L1 hi B cells saw attenuated Ig production ( Fig. 2a ) and T FH -cell expansion ( Fig. 2b ) in a dose-dependent manner, suggesting that the proportion of PD-L1 hi B cells may regulate humoral responses. Mice that only received PD-L1 lo / int B cells were assessed to ensure that there were no PD-L1 hi cells present before immunization ( Supplementary Fig. 4c ). Animals that were devoid of PD-L1 hi B cells demonstrated a significant expansion in the proportion and number of T FH cells in the spleen ( Fig. 2h ) and ( Fig. 2i ), while B-cell-deficient mice that were reconstituted with a homoeostatic level (~5%) of PD-L1 hi B cells demonstrated T FH expansion on par with immunized WT animals. This suggests that a ‘natural’ population of PD-L1 hi B cells is primarily responsible for homoeostatic regulation of T FH cells and the subsequent humoral response. Alternative modes of T FH -cell regulation are not required As described earlier ( Supplementary Fig. 3 ), PD-L1 hi B cells were found to express significantly less IL-10 compared with all other PD-L1-expressing B-cell subsets. IL-10 secreting Breg cells have been described by Tedder [1] , [3] , [30] and others [23] , [31] . Interestingly, Tedder and co-workers [30] have described how IL-10-producing B cells utilize IL-21, a key T FH cytokine, as part of their maintenance. To address whether IL-10 contributed to the suppressive activity of PD-L1 hi B cells on T FH -cell expansion PD-L1 hi B cells were adoptively transferred from WT and Il10 −/− mice into KLH/CFA-immunized WT and Pdl1 −/− animals. Upon transfer, there was no difference in the suppressive activity between WT-PD-L1 hi and Il10 −/− -PD-L1 hi B cells ( Supplementary Fig. 5a,b ). This suggests that the suppression of T FH cells by PD-L1 hi B cells is not IL-10 mediated. We, and others, have previously demonstrated that a Breg population can drive FoxP3 regulatory T cells (T REG ) through IL-10 secretion [23] . Transfer of PD-L1 hi B cells into WT mice did not alter the frequency and proportion of T REG (defined as CD4 + FoxP3 + ) in the dLN ( Supplementary Fig. 5c ). We therefore addressed whether PD-L1 hi B cells could evoke a T REG response, secondary to adoptive transfer. To address the role of T REG cells in PD-L1 hi B-cell-mediated regulation of T FH cells, DEREG mice (which express a diphtheria toxin (DT) receptor–enhanced green fluorescent protein fusion protein under the control of the foxp3 gene locus, allowing selective depletion of FoxP3 + T REG cells by DT injection [32] ) were used. Depletion was confirmed by flow cytometry ( Supplementary Fig. 5d ). As demonstrated by Vaeth et al . [33] , immunization of DT-treated animals demonstrated increased T FH -cell expansion in both the spleen and dLN ( Supplementary Fig. 5e ). WT mice were treated with DT only and were found to have no change in the proportion or number of T FH cells on immunization. Adoptive transfer of 1 × 10 6 PD-L1 hi B cells into DT-treated, KLH/CFA-immunized mice attenuated T FH expansion in the spleen and dLN. The recent identification of T FR cells (defined as CD4 + B220 − CXCR5 + PD-1 + FoxP3 + ) has provided elegant insight into the homoeostatic control of the humoral response [17] , [18] , [34] . Transfer of PD-L1 hi B cells significantly reduced the proportion and number of T FR cells in the spleen and dLN ( Supplementary Fig. 6a ). Assessment of T FR cells from immunized Pdl1 −/− animals demonstrated a significantly elevated proportion and number in the spleen and dLN ( Supplementary Fig. 6b,c ). These findings are in agreement with recent studies by Sage et al . [18] , who note that PD-L1 ligation restricts T FR -cell activity in the dLN. We also investigated the presence of CD8 + T REG cells (defined as CD8 + CXCR5 hi CD44 hi CD122 hi ), which have been previously reported to be important in self-tolerance and T FH expansion [19] . On KLH/CFA immunization and PD-L1 hi B-cell adoptive transfer there was no expansion in CD8 + T REG cells, suggesting that they also are not involved in PD-L1 hi B-cell-mediated T FH -cell suppression ( Supplementary Fig. 6b ). These results indicate that PD-L1 hi B cells act as a Breg with elevated expression of PD-L1 being critical for suppressive activity. Interestingly, these cells function independent of IL-10 production, suggesting an alternative means of Breg activity. T REG - (both CD4 + and CD8 + ) or TFR-cell induction was also not required to elicit a suppressive effect, suggesting a direct mode of action. PD-L1 hi B-cell adoptive transfer suppresses EAE B cells are known to have paradoxical roles in autoimmune disease with regulatory [30] , [31] , [35] and effector [36] functions. One of the predominant drivers of auto-reactive B cells are T FH cells, and given the plethora of data on elevated T FH cells in autoimmune disease [20] it stands that PD-L1 hi B cells may have a critical role in regulating aberrant autoimmune responses. Experimental autoimmune encephalomyelitis (EAE) was employed as a disease model. Mice received PD-L1 hi B cells either 7 days before (D−7) or 7 days after (D+7) immunization with the encephalitogenic peptide from myelinoligodendrocyte glycoprotein in CFA (MOG 35–55 /CFA) ( Fig. 3a ). 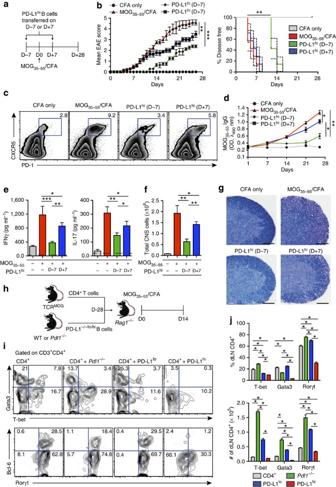Figure 3:PD-L1hiB cells suppress EAE. (a) EAE was induced in wild-type animals. Groups were either CFA-alone (grey line, circle;n=6), MOG35–55/CFA immunized at D0 (red line, triangle;n=8), received PD-L1hiB cells 7 days before (D−7) immunization (green line, diamond;n=7) or received PD-L1hiB cells 7 days after (D+7) immunization (blue line, square;n=7). (b) Clinical EAE score (mean±s.e.m.) and disease-free interval (mean±s.e.m.) demonstrate PD-L1hiB-cell transfer can reduce disease severity and onset. Cumulative disease scores were compared using two-tailed unpairedt-test. Disease-free intervals were compared using Wilcoxon test. (c) Analysis of dLN for TFHcells at Day 14 via flow cytometry. (d) Production of MOG35–55-specific IgG was assessed over the course of EAE via ELISA. (e) dLN were collected from mice on Day 26 after EAE induction, and re-stimulated individually for 72 h with 10 μg ml−1MOG35–55. Supernatants were analyzed by ELISA to determine concentrations of IFN-γ and IL-17. (f) Spinal cord cell infiltrates were assessed at Day 14 using Trypan Blue. (g) Spinal cord histology, Luxol-Fast/eosin-stained sections of spinal cord at Day 14. Scale bar, 100 μm. (h) TCRMOGCD4+cells and either PD-L1−/−/lo/hiB cells were transferred intoRag1−/−mice and immunized with MOG35–55for 14 days. (i) Flow cytometry analysis of CD4+T cells for T-bet, Gata3 and Bcl-6 and Rorγt. (j) Quantification of CD4+T-cell differentiation via flow cytometry. Representative plots and images are shown. Data show representative results from two independent experiments (error bars, s.e.m.). For adoptive transfer experiments intoRag1−/−animals, six mice per group were used. *P<0.05, **P<0.01 and ***P<0.001 (Student’st-test). Figure 3: PD-L1 hi B cells suppress EAE. ( a ) EAE was induced in wild-type animals. Groups were either CFA-alone (grey line, circle; n=6 ), MOG 35–55 /CFA immunized at D0 (red line, triangle; n=8 ), received PD-L1 hi B cells 7 days before (D−7) immunization (green line, diamond; n=7 ) or received PD-L1 hi B cells 7 days after (D+7) immunization (blue line, square; n=7 ). ( b ) Clinical EAE score (mean±s.e.m.) and disease-free interval (mean±s.e.m.) demonstrate PD-L1 hi B-cell transfer can reduce disease severity and onset. Cumulative disease scores were compared using two-tailed unpaired t -test. Disease-free intervals were compared using Wilcoxon test. ( c ) Analysis of dLN for T FH cells at Day 14 via flow cytometry. ( d ) Production of MOG 35–55 -specific IgG was assessed over the course of EAE via ELISA. ( e ) dLN were collected from mice on Day 26 after EAE induction, and re-stimulated individually for 72 h with 10 μg ml −1 MOG 35–55 . Supernatants were analyzed by ELISA to determine concentrations of IFN-γ and IL-17. ( f ) Spinal cord cell infiltrates were assessed at Day 14 using Trypan Blue. ( g ) Spinal cord histology, Luxol-Fast/eosin-stained sections of spinal cord at Day 14. Scale bar, 100 μm. ( h ) TCR MOG CD4 + cells and either PD-L1 −/−/lo/hi B cells were transferred into Rag1 −/− mice and immunized with MOG 35–55 for 14 days. ( i ) Flow cytometry analysis of CD4 + T cells for T-bet, Gata3 and Bcl-6 and Rorγt. ( j ) Quantification of CD4 + T-cell differentiation via flow cytometry. Representative plots and images are shown. Data show representative results from two independent experiments (error bars, s.e.m.). For adoptive transfer experiments into Rag1 −/− animals, six mice per group were used. * P <0.05, ** P <0.01 and *** P <0.001 (Student’s t -test). Full size image MOG-immunized mice developed EAE which was significantly attenuated in mice receiving PD-L1 hi B cells on D−7 as well as when cells were transferred on D+7. Furthermore, mice receiving PD-L1 hi B cells at both time points had significantly delayed disease onset relative to control mice ( Fig. 3b ). The reduced disease in MOG-primed recipients of PD-L1 hi B cells was associated with a significant reduction in T FH -cell generation at Day 14 after immunization ( Fig. 3c ). In addition to this, the reduction in T FH cells in recipients of PD-L1 hi B cells resulted in a significantly concomitant decrease in MOG 35–55 -specific IgG ( Fig. 3d ). The timing of cell transfer is crucial to the influence on disease progression as animals receiving PD-L1 hi B cells at D+7 failed to arrest disease onset but did reduce disease severity ( Fig. 3b ), with greater levels of T FH cells ( Fig. 3c ) and MOG 35–55 -specific IgG in comparison to recipients of PD-L1 hi B cells at D−7 ( Fig. 3d ). EAE pathogenesis involves Th1 and Th17 cells, which express interferon-gamma (IFN-γ) and IL-17, respectively [37] , [38] , that infiltrate the CNS [39] . PD-L1 hi B-cell recipients displayed a significant decrease in MOG-specific production of IFN-γ and IL-17 from dLN cells compared with control mice ( Fig. 3e ). There was significantly decreased CNS cell infiltration ( Fig. 3f ), which was validated by histological examination of spinal cord tissue ( Fig. 3g ), in PD-L1 hi B-cell recipients irrespective of the time of administration. The transfer of PD-L1 hi B cells did not increase the proportion of T REG ( Supplementary Fig. 5c ), which are known to be protective in EAE [40] , suggesting that PD-L1 hi B cells limited disease by reducing the accumulation of pathogenic cells at the target organ. PD-L1 hi B cells were not found in the spinal cord, indicating a systemic role, rather than effects at the site of inflammation. To further decipher the cellular mechanisms underlying the suppressive activities of PD-L1 hi B cells in EAE, we adoptively transferred TCR MOG CD4 + T cells either alone or with Pdl1 −/− B cells or PD-L1 lo or PD-L1 hi B cells from WT mice into Rag1 −/− animals before immunizing with MOG 35–55 /CFA ( Fig. 3h ). Fourteen days later dLNs were recovered and CD4 + T cells were analyzed for expression of the common T-cell subset transcription factors (Th1; T-bet, Th2; Gata3, Th17/T FH ; Rorγt and T FH ; Bcl-6) via flow cytometry ( Fig. 3i ). Recipients of PD-L1 hi B cells demonstrated a significant downregulation in both the proportion and number of T-bet + , Gata3 + and Rorγt + CD4 + T cells (Bcl-6 + were not enumerated due to their overlap with Rorγt + CD4 + T cells [6] ). This suggests that PD-L1 hi B cells can influence in vivo T-cell differentiation. PD-L1 hi B cells restrict T-cell differentiation Having established that PD-L1 hi B cells can directly suppress T-cell responses we sought to address how this process occurred. CD4 + T cells and B220 + B cells were isolated from WT mice and stimulated with the bacterial superantigen Staphylococcus enterotoxin B (SEB) for 5 days. After co-culture, a proportion of CD4 + T cells became CXCR5 + PD-1 + and expressed the transcription factor Bcl-6 ( Fig. 4a ). CD4 + T cells were stimulated with SEB in the presence of PD-L1 lo , PD-L1 int or PD-L1 hi expressing B-cell subsets. CD4 + T cells co-cultured with PD-L1 hi B cells had significantly reduced expansion of CD4 + CXCR5 + PD-1 + Bcl-6 + cells compared with those cultured with PD-L1 lo or PD-L1 int B cells ( Supplementary Fig. 7a ). There were also significant decreases in IL-21 and IgG production ( Supplementary Fig. 7b ). These results indicate that PD-L1 hi B cells can suppress T FH -cell differentiation in vitro . 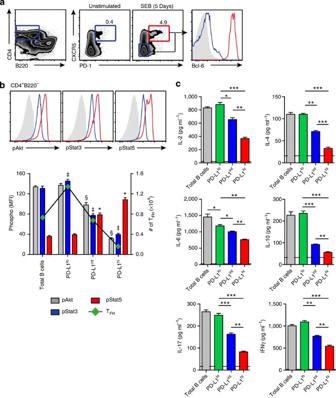Figure 4:PD-L1hiB cells restrict T-cell differentiation. (a) Co-cultures of CD4+T cells and CD19+B cells were stimulated with 1 μg ml−1SEB for 5 days and then analyzed via flow cytometry for CD4+B220−cells that expressed CXCR5, PD-1 and Bcl-6. These were defined as TFHcells (b) Graph depicting the correlation between phospho-Akt (pAkt), phospho-Stat3 (pStat3), phospho-Stat5 (pStat5) and number of TFHcells in co-cultures of SEB-stimulated CD4+T cells with PD-L1lo/int/hiB cells. § denotes significance (P<0.05) of pAkt, ‡ denotes significance (P<0.05) of pStat3 and * denotes significance (P<0.05) of pStat5 between groups (c) Analysis of co-culture supernatant for IL-2, IL-4, IL-6, IL-10, IL-17 and IFNγ via ELISA. Representative plots are shown. *P<0.05, **P<0.001 and ***P<0.0001 (Student’st-test). Data are representative of four experiments run in quadruplicate (error bars, s.e.m.). Figure 4: PD-L1 hi B cells restrict T-cell differentiation. ( a ) Co-cultures of CD4 + T cells and CD19 + B cells were stimulated with 1 μg ml −1 SEB for 5 days and then analyzed via flow cytometry for CD4 + B220 − cells that expressed CXCR5, PD-1 and Bcl-6. These were defined as T FH cells ( b ) Graph depicting the correlation between phospho-Akt (pAkt), phospho-Stat3 (pStat3), phospho-Stat5 (pStat5) and number of T FH cells in co-cultures of SEB-stimulated CD4 + T cells with PD-L1 lo/int/hi B cells. § denotes significance ( P <0.05) of pAkt, ‡ denotes significance ( P <0.05) of pStat3 and * denotes significance ( P<0.05 ) of pStat5 between groups ( c ) Analysis of co-culture supernatant for IL-2, IL-4, IL-6, IL-10, IL-17 and IFNγ via ELISA. Representative plots are shown. * P <0.05, ** P <0.001 and *** P <0.0001 (Student’s t -test). Data are representative of four experiments run in quadruplicate (error bars, s.e.m.). Full size image Given the propensity of PD-L1 hi B cells to suppress T-cell responses, we investigated how this occurs following PD-1 ligation. Akt signalling is essential for naive T-cell activation and proliferation and has been shown previously to be downregulated upon PD-1 ligation [14] . Furthermore, recent work on the dynamic regulation of not only T FH cells [41] , but also Th1 (ref. 42 ) and Th17 (refs 43 , 44 ) has described critical roles for Stat3 (refs 6 , 45 , 46 ) and Stat5 (ref. 47 ) in terms of both induction and suppression, respectively. Therefore the effects of PD-L1 hi B cells on T-cell differentiation through PD-1 ligation were studied with respect to phosphorylation of Akt (pAkt), Stat3 (pStat3) and Stat5 (pStat5) following T-cell activation in vitro. CD4 + T cells, co-cultured with PD-L1 hi B cells, exhibited significantly increased expression of pStat5 with a concomitant decrease in pAkt and pStat3 ( Fig. 4b ). Conversely, T cell co-cultures with PD-L1 lo or PD-L1 int B cells expressed elevated pAkt and pStat3 with lower expression of pStat5 ( Fig. 4b ). When correlating the number of T FH cells in culture with pAkt, pStat3 and pStat5 expression, we found, as previously reported [47] , that pStat5 expression was inversely proportional to T FH -cell differentiation while pAkt and pStat3 levels were positively correlative. Crucially, co-cultures with PD-L1 lo B cells exhibited the highest levels of pAkt and pStat3, suggesting that suppression of T FH -cell differentiation was dependent on PD-L1 hi B cells. To further confirm that PD-L1 hi B-cell regulation of T-cell differentiation was via the PD-1/PD-L1/PD-L2 pathway we used our co-culture system in the presence or absence of blocking mAbs to PD-L1, PD-L2 and PD-1 ( Supplementary Fig. 7c ). Blockade of PD-L1 and/or PD-1 both drove significant decreases in pStat5 and increases in pAkt and pStat3 levels within CD4 + T cells. To further validate the effects of PD-L1 hi B cells on T-cell activation and differentiation, co-culture supernatants were analyzed for, in addition to IL-21 ( Supplementary Fig. 7b ), IL-2, IL-4, IL-6, IL-10, IL-17 and IFN-γ ( Fig. 4c ). Co-cultures with PD-L1 hi B cells demonstrated significantly reduced levels of the above cytokines, suggesting attenuation of the T-cell response to stimuli. This data suggests that PD-L1 hi B cells regulate T-cell differentiation via alterations in downstream signalling pathways following PD-1 ligation. Residual B cells post αCD20 mAb treatment are PD-L1 hi Rituximab (RTX), an αCD20 antibody, is used to manage and treat B-cell malignancies as well as autoimmune disorders such as rheumatoid arthritis [48] . Although first considered to deplete autoantibody producing plasma cells, B-cell depletion therapy appears to have a multi-faceted mode of action [49] . We sought to investigate if B-cell depletion therapy influenced PD-L1 hi B cells. The B-cell depletion kinetics of WT mice were monitored over 45 days, following αCD20 mAb treatment. Post treatment, up to 90% of CD3 − CD19 + cells were depleted in the blood after 3 days ( Fig. 5a ) with 75% depletion in the spleen seen within 9 days, as reported elsewhere [49] , [50] , [51] . Interestingly, as the total number and proportion of CD3 − CD19 + cells decreased, the percentage of PD-L1 hi CD3 − CD19 + B cells, as a proportion of total CD3 − CD19 + cells, significantly increased ( Fig. 5b ). Throughout the 45-day course, the proportion of PD-L1 hi CD3 − CD19 + B cells that made up the total B-cell compartment was significantly increased ( Fig. 5b ). Crucially, the number of these cells did not change throughout the treatment course. 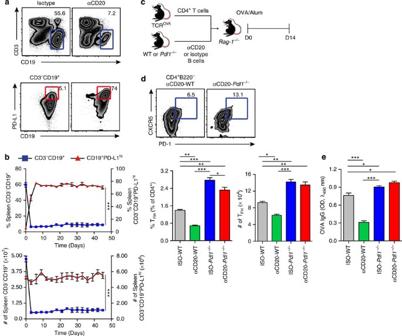Figure 5:PD-L1hiB cells are refractory to αCD20 mAb treatment. (a) Flow cytometry analysis of CD3−CD19+PD-L1hiB-cell populations within the spleens of mice 8 days after receiving either isotype or αCD20 treatment. (b) Quantification of the proportion of CD3−CD19+PD-L1hiB cells post treatment over 45 days. (c) B cells (4 × 106) from wild-type (WT) (which have received either isotype (ISO-WT) or αCD20 mAb (αCD20-WT) orPdl1−/−mice (ISO-Pdl1−/−; αCD20-Pdl1−/−)) were co-transferred with TCROVACD4+T cells intoRag1−/−animals. (d) Quantification of TFHcells in the dLN via flow cytometry of OVA-immunized mice that had received either αCD20-WT B cells or αCD20-Pdl1−/−B cells. (e) OVA-specific total IgG production was analyzed via ELISA. Representative plots are shown. *P<0.05, **P<0.001 and ***P<0.0001 (Student’st-test). Data are representative of two experiments with four mice per group (error bars, s.e.m.). Figure 5: PD-L1 hi B cells are refractory to αCD20 mAb treatment. ( a ) Flow cytometry analysis of CD3 − CD19 + PD-L1 hi B-cell populations within the spleens of mice 8 days after receiving either isotype or αCD20 treatment. ( b ) Quantification of the proportion of CD3 − CD19 + PD-L1 hi B cells post treatment over 45 days. ( c ) B cells (4 × 10 6 ) from wild-type (WT) (which have received either isotype (ISO-WT) or αCD20 mAb (αCD20-WT) or Pdl1 −/− mice (ISO- Pdl1 −/− ; αCD20- Pdl1 −/− )) were co-transferred with TCR OVA CD4 + T cells into Rag1 −/− animals. ( d ) Quantification of T FH cells in the dLN via flow cytometry of OVA-immunized mice that had received either αCD20-WT B cells or αCD20- Pdl1 −/− B cells. ( e ) OVA-specific total IgG production was analyzed via ELISA. Representative plots are shown. * P <0.05, ** P <0.001 and *** P <0.0001 (Student’s t -test). Data are representative of two experiments with four mice per group (error bars, s.e.m.). Full size image This led us to investigate whether αCD20 mAb therapy left a residual PD-L1 hi B-cell population that suppressed T-cell responses. To study the activity of these residual post αCD20 mAb PD-L1 hi B cells, CD4 + T cells from OT-II mice (which possess an ovalbumin (OVA)-specific TCR) were co-transferred with B cells from WT (CD20-WT) or Pdl1 −/− (CD20- Pdl1 −/− ) animals that had either received αCD20 mAb therapy or an isotype control (ISO) into Rag1 −/− recipients ( Fig. 5c ). Mice were allowed to reconstitute before being immunized subcutaneously in the footpad with an OVA/alum mixture. Recipients of CD20- Pdl1 −/− B cells exhibited a significant T FH -cell expansion compared with recipients of CD20-WT B cells ( Fig. 5c ). OVA-specific IgG was also significantly elevated ( Fig. 5d ). Interestingly, ISO-WT B-cell recipients also demonstrated significant T FH -cell expansion, compared with CD20-WT B-cell recipients ( Fig. 5b ), suggesting that the B cells from the CD20-WT were potent suppressors of T-cell proliferation and differentiation. Together, these observations indicate that αCD20 mAb therapy generates a residual B-cell population that is PD-L1 hi and such cells have potent T-cell-suppressive activity. It also demonstrates that these PD-L1 hi B cells require PD-L1 to elicit a suppressive effect. PD-L1 hi B cells use BAFF to survive αCD20 treatment To determine how PD-L1 hi B cells are a residual population following αCD20 mAb therapy, we sought to investigate the role of B-cell-specific survival factors. The TNF family ligands APRIL (CD256 and TNFSF13) and BAFF (also known as BLyS, TALL-1, CD257 and TNFSF13B) are known to support B-cell survival [52] . These factors interact with three TNFR family members, TACI (CD267 and TNFRSF13B), BAFF-R (also known as BR3, CD268 or TNFRSF17) and BCMA (CD269 and TNFRSF13C) with differing affinities [53] , with BAFF-R and TACI demonstrating the highest affinity for BAFF and APRIL, respectively [54] . Interestingly, studies from various groups have demonstrated an elevation in BAFF [54] , [55] , [56] , but not APRIL [57] , post αCD20 mAb therapy. Analysis of murine serum post αCD20 therapy demonstrated significantly elevated levels of BAFF ( Fig. 6a ). 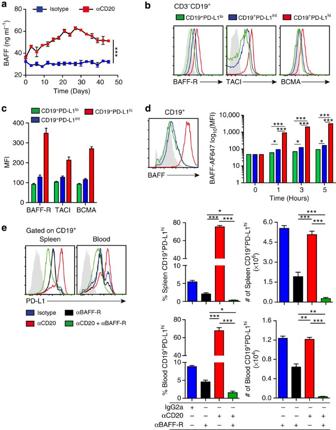Figure 6:PD-L1hiB cells act as BAFF ‘sinks’. (a) Serum BAFF levels, measured via ELISA, in mice treated with αCD20 mAb. (b) Expression of BAFF receptors BAFF-R, TACI and BCMA were correlated to PD-L1 B-cell expression via flow cytometry (PD-L1lo(green), PD-L1int(blue) and PD-L1hi(red)). Histograms are representative of six mice. (c) Flow cytometry analysis of BAFF-R, TACI and BCMA on PD-L1-expressing B-cell subsets 8 days after αCD20 mAb treatment. (d) To demonstrate functional significance, BAFF was conjugated to a fluorochrome (AF647) and administered (0, 0.01, 0.1, 1, 10, 100 and 1,000 ng ml−1) to whole B-cell culturesin vitro. Cells were analyzed via flow cytometry at 0, 1, 3 and 5 h to detected AF647 association with PD-L1-expressing B-cell subsets (PD-L1lo(green), PD-L1int(blue) and PD-L1hi(red)). (e) Quantification of PD-L1hiB cells via flow cytometry in the blood and spleen following αBAFF-R mAb treatment alone or in combination with αCD20 mAbin vivo(e). Representative plots are shown. *P<0.05, **P<0.001 and ***P<0.0001 (Student’st-test). Data are representative of two experiments with six mice per group (error bars, s.e.m.). Figure 6: PD-L1 hi B cells act as BAFF ‘sinks’. ( a ) Serum BAFF levels, measured via ELISA, in mice treated with αCD20 mAb. ( b ) Expression of BAFF receptors BAFF-R, TACI and BCMA were correlated to PD-L1 B-cell expression via flow cytometry (PD-L1 lo (green), PD-L1 int (blue) and PD-L1 hi (red)). Histograms are representative of six mice. ( c ) Flow cytometry analysis of BAFF-R, TACI and BCMA on PD-L1-expressing B-cell subsets 8 days after αCD20 mAb treatment. ( d ) To demonstrate functional significance, BAFF was conjugated to a fluorochrome (AF647) and administered (0, 0.01, 0.1, 1, 10, 100 and 1,000 ng ml −1 ) to whole B-cell cultures in vitro . Cells were analyzed via flow cytometry at 0, 1, 3 and 5 h to detected AF647 association with PD-L1-expressing B-cell subsets (PD-L1 lo (green), PD-L1 int (blue) and PD-L1 hi (red)). ( e ) Quantification of PD-L1 hi B cells via flow cytometry in the blood and spleen following αBAFF-R mAb treatment alone or in combination with αCD20 mAb in vivo ( e ). Representative plots are shown. * P <0.05, ** P <0.001 and *** P <0.0001 (Student’s t -test). Data are representative of two experiments with six mice per group (error bars, s.e.m.). Full size image Subsequently, we investigated the expression profile of BAFF-R, TACI and BCMA on PD-L1-expressing B-cell subsets ( Fig. 6b ). We found that PD-L1 hi B cells expressed the highest amount of BAFF-R, TACI and BCMA, compared with PD-L1 lo and PD-L1 int B cells. Crucially, PD-L1 hi B cells from αCD20 mAb-treated mice, also expressed elevated BAFF-R, TACI and BCMA ( Fig. 6c ). This suggested that PD-L1 hi B cells have the propensity to sequester BAFF from the milieu and thus promote their survival, especially in a B-cell depleted environment. To demonstrate this phenomena, we conjugated BAFF to a fluorochrome (BAFF–AF647) and added it in a dose-dependent manner (0, 1, 10, 100, 1,000 ng ml −1 ) to B220 + B cells in vitro and assessed BAFF–AF647 + binding to PD-L1 lo/int/hi B cells at 0, 1, 3 and 5 h ( Fig. 6d ). PD-L1 hi B cells demonstrated the greatest degree of BAFF–AF647 association at all time points ( Fig. 6d ), in agreement with the preferential expression of BAFF-R on PD-L1 hi B cells ( Fig. 6b ). This data indicates that PD-L1 hi B cells preferentially sequester BAFF in comparison to other PD-L1 B-cell-expressing subsets. To understand whether this BAFF sequestration by PD-L1 hi B cells was BAFF-R mediated and of functional significance, we treated WT mice with αCD20 mAb and monitored serum BAFF levels. At Day 8 (when CD19 + B220 + B-cell counts are at their lowest and proportion of PD-L1 hi B cells are at their highest, Fig. 5a ), αBAFF-R mAb was administered to block BAFF/BAFF-R interactions. On analysis, we found that BAFF-R blockade enhanced PD-L1 hi B-cell sensitivity to αCD20 mAb therapy with subsequent depletion of these cells ( Fig. 6e ), suggesting a role for BAFF in the resistance of PD-L1 hi B cells to depletion. Human B cells require PD-L1 to restrict cT FH -cell expansion Finally, we explored whether PD-L1 expression on human circulating B cells had an influence on T FH -cell activity. Recently, circulating CD4 + CXCR5 + ‘T FH -like’ cells and lymphoid organ-resident T FH cells have been delineated [11] , [12] , [58] . We defined circulating human T FH (cT FH ) cells as CD4 + CXCR5 + PD-1 + ( Supplementary Fig. 8a ). Furthermore, cT FH also expressed ICOS and BCL-6, when detected in both peripheral blood mononuclear cells ( Supplementary Fig. 8a ). To determine whether PD-L1 was involved in regulating circulating T-cell responses, and in particular circulating T FH -cell responses, we stimulated whole blood from healthy volunteers with SEB for 3 days leading to the generation of a population of cT FH cells ( Fig. 7a ). Using an αPD-L1 blocking antibody there was a significant increase in the proportion and number of cT FH in a dose-dependent manner in blood ( Fig. 7a ), demonstrating the importance of PD-L1 expression with regards to regulation of circulating T-cell proliferation and differentiation. In addition, there were concordant changes in IL-6, IL-21 and IgG production ( Supplementary Fig. 8b ). 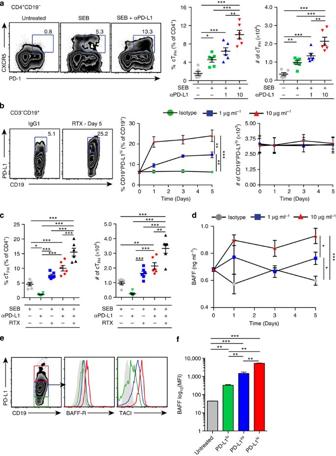Figure 7:PD-L1 on human B cells is a crucial regulator of cTFHcells. (a) Flow cytometry analysis of cTFHcells from heparinized whole blood from healthy volunteers after stimulation with 1 μg ml−1SEB in the presence or absence of either 1 μg ml−1or 10 μg ml−1αPD-L1 mAb. (b) Quantification of CD3−CD19+PD-L1hicells followingex vivodepletion of B cells using 1 or 10 μg ml−1Rituximab (RTX) over 5 days (c) Quantification of cTFHcells from SEB-stimulated whole blood in the presence or absence or combination of RTX and αPD-L1 treatment. (d) BAFF concentration of RTX-treated whole blood as measured via ELISA. (e) Expression of BAFF-R and TACI were correlated to PD-L1 B-cell expression via flow cytometry (PD-L1lo(green), PD-L1int(blue) and PD-L1hi(red)). (f) To demonstrate functional significance, BAFF was conjugated to a fluorochrome (AF647) and administered (0, 0.01, 0.1, 1, 10, 100 and 1,000 ng ml−1) to whole B-cell culturesin vitro. Cells were analyzed at 0, 1, 3 and 5 h to detect AF647 association with PD-L1-expressing B-cell subsets via flow cytometry (PD-L1lo(green), PD-L1int(blue) and PD-L1hi(red)). Representative plots are shown. *P<0.05, **P<0.001 and ***P<0.0001 (Student’st-test). Data are representative of six samples with experiments run in triplicate (error bars, s.e.m.). Figure 7: PD-L1 on human B cells is a crucial regulator of cT FH cells. ( a ) Flow cytometry analysis of cT FH cells from heparinized whole blood from healthy volunteers after stimulation with 1 μg ml −1 SEB in the presence or absence of either 1 μg ml −1 or 10 μg ml −1 αPD-L1 mAb. ( b ) Quantification of CD3 − CD19 + PD-L1 hi cells following ex vivo depletion of B cells using 1 or 10 μg ml −1 Rituximab (RTX) over 5 days ( c ) Quantification of cT FH cells from SEB-stimulated whole blood in the presence or absence or combination of RTX and αPD-L1 treatment. ( d ) BAFF concentration of RTX-treated whole blood as measured via ELISA. ( e ) Expression of BAFF-R and TACI were correlated to PD-L1 B-cell expression via flow cytometry (PD-L1 lo (green), PD-L1 int (blue) and PD-L1 hi (red)). ( f ) To demonstrate functional significance, BAFF was conjugated to a fluorochrome (AF647) and administered (0, 0.01, 0.1, 1, 10, 100 and 1,000 ng ml −1 ) to whole B-cell cultures in vitro . Cells were analyzed at 0, 1, 3 and 5 h to detect AF647 association with PD-L1-expressing B-cell subsets via flow cytometry (PD-L1 lo (green), PD-L1 int (blue) and PD-L1 hi (red)). Representative plots are shown. * P <0.05, ** P <0.001 and *** P <0.0001 (Student’s t -test). Data are representative of six samples with experiments run in triplicate (error bars, s.e.m.). Full size image PD-L1 expression on human B cells was also assessed, with a proportion of PD-L1 hi B cells observed, suggesting similarities with the population found in mice. Phenotypic analysis of human PD-L1 hi B cells suggested that the majority of these cells have a naïve B-cell phenotype (CD19 + CD10 − CD21 + CD27 − ; Supplementary Fig. 8c ). To correlate our findings in mice with those in man, we depleted B cells in whole blood from healthy volunteers ex vivo using the human αCD20 mAb (RTX). Treatment of whole blood with RTX exhibited efficient >90% B-cell depletion over 5 days of culture ( Supplementary Fig. 8d ). After 1 day, post treatment, a population of B cells that expressed PD-L1 hi was detectable ( Fig. 7b ). As seen in mice, the number of PD-L1 hi B cells was unchanged, post-RTX treatment. We next investigated whether this residual population of PD-L1 hi B cells could restrict cT FH -cell generation. Whole blood from healthy donors was treated with a combination of RTX and SEB, with or without the presence of αPD-L1 blocking mAb. Groups treated with RTX, SEB and αPD-L1 exhibited higher cT FH cells compared with those treated with RTX and SEB ( Fig. 7c ). BAFF concentrations in whole-blood cultures were evaluated and, as per recent reports [54] , [55] , [57] , were elevated post-RTX treatment ( Fig. 7d ). The elevated levels of BAFF, post-RTX treatment, would suggest that human PD-L1 hi B cells are refractory to depletion in a similar way to their murine counterparts via elevated BAFF-R expression. Indeed, PD-L1 high expressing human B cells also expressed the highest level of BAFF-R ( Fig. 7e ). To assess the functional nature of this expression, CD19 + B cells were cultured in the presence of fluorochrome-conjugated BAFF. As demonstrated earlier in mice, human CD19 + PD-L1 hi B cells exhibited the highest association with BAFF ( Fig. 7f ). Together, these results demonstrate the existence of a PD-L1 hi B-cell population in man that can suppress cT FH -cell expansion and is refractory to B-cell depletion therapy. The mechanisms that regulate T FH -cell activity are only beginning to be elucidated. The immune regulatory functions of T FR cells have only recently been described [17] , [18] , [34] , yet little is known about the regulatory role B cells have on T FH responses. The majority of studies on Breg cells have focused on their predisposition to produce IL-10 and suppress in a range of autoimmune or allergic conditions in both mice and man [22] . In this study, we have identified a previously unknown function of Breg cells that requires PD-L1 hi to regulate T FH -cell expansion and differentiation and suppress autoimmune disease. We have previously shown [16] , and demonstrated here, that absence of PD-L1 on B cells led to elevated T FH cells with abundant IgG production. Investigating the abundance of PD-L1 on B cells led to the identification of a high expressing subset in both lymphoid organs and the blood. This suggested that these PD-L1 hi B cells might have a greater suppressive effect on T FH responses, compared with lower expressing subsets. The PD-1 pathway acts on many parts of the immune response; however, biological complexity has led to inconsistencies about the role of this pathway in humoral immunity [15] , [59] . Our adoptive transfer studies of PD-L1 hi B cells demonstrated their potency at suppressing T FH activity. Crucially, we have been able to demonstrate that a lack of these cells leads to increased T FH responses. On transfer of homoeostatic numbers of PD-L1 hi B cells, T FH -cell activity returns to a basal level, suggesting that this subset of cells is required for normal regulation of the humoral response. We also determined that PD-L1 hi B cells utilized PD-L1 as its main suppressive mechanism. IL-10, a well-characterized means of B-cell-mediated immune suppression [22] , [30] , was not required for PD-L1 hi B-cell-suppressive activity. Furthermore, T REG cells were not required for PD-L1 hi B-cell-mediated suppression, suggesting a direct interaction with target T cells. PD-L1 hi B cells did reduce the proportion of T FR cells. However, as elegantly described by Sage et al . [18] , the change in proportion or number of T FR cells is not critical but rather the ratio to T FH cells governs their suppressive activity. Using the EAE model we show that PD-L1 hi B cells are suppressive in vivo . Following transfer to MOG-primed mice, recipients of PD-L1 hi B cells delayed the onset and severity of disease. Amelioration of EAE by PD-L1 hi B cells was associated with reduced T FH -cell expansion and the generation of MOG 35–55 -specific IgG, as well as reduced production of antigen-induced IL-17 and IFN-γ. Analysis of CD4 + T-cell subsets in recipients of PD-L1 hi B cells indicates a broad range of suppressive targets, rather than just T FH cells as other previously defined Breg cells have also demonstrated [3] , [60] , [61] . This lends itself to the hypothesis that ligation of the PD-1 pathway may modulate T-cell differentiation. As PD-L1 hi B cells can also be detected in the periphery, it is possible that these cells can restrict circulating T cells. The amalgamation of signals through inhibitory receptors such as PD-1, activation of TCRs and ligation of cytokine receptors may alter the differentiation of various T-cell subsets [62] . Through both in vivo and in vitro studies, we are able to show that PD-L1 hi B cells could restrict T-cell differentiation, which is partially caused by an upregulation of Stat5, a known suppressor of T FH generation [47] , [63] and also known to affect Th1 and Th17 responses. Therefore, our studies suggest that PD-L1 hi B cells have broader implications than just a suppressive role in the differentiation of T FH cells ( Fig. 8 ). The T REG -independent effect of PD-L1 hi B cells on effector T-cell subsets is demonstrative of a novel B-cell-mediated suppressive mechanism. As PD-L1 interactions have been shown to modulate T REG (ref. 64 ) and T FR (ref. 18 ) cell activity, it could be reasoned that PD-L1 hi B cells alter the effector/regulatory T-cell ratio, thus limiting T-cell effector function. Further studies are required to delineate the interplay between effector T-cell subsets and PD-L1 hi B cells. 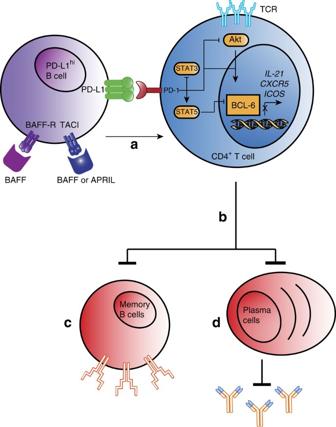Figure 8: Model for PD-L1hiB-cell function. PD-L1hiB cells (which express higher levels of BAFF-R and TACI) interact with PD-1 on activated T cells (a). For TFH-cell differentiation, activation of Akt and Stat3 lead to increased transcription of Bcl-6. Interactions with PD-L1hiB cells cause an increase in Stat5 expression, a known suppressor of TFH-cell development and expansion (b). A reduction in TFHcells limits B-cell fate by limiting both memory B-cell development (c) and terminal differentiation to plasma cells (d). Figure 8: Model for PD-L1 hi B-cell function. PD-L1 hi B cells (which express higher levels of BAFF-R and TACI) interact with PD-1 on activated T cells ( a ). For T FH -cell differentiation, activation of Akt and Stat3 lead to increased transcription of Bcl-6. Interactions with PD-L1 hi B cells cause an increase in Stat5 expression, a known suppressor of T FH -cell development and expansion ( b ). A reduction in T FH cells limits B-cell fate by limiting both memory B-cell development ( c ) and terminal differentiation to plasma cells ( d ). Full size image We sought to understand the therapeutic relevance of this discovery by looking at the role of RTX therapy on PD-L1 hi B cells. Despite efficient B-cell depletion in mice, PD-L1 hi B cells were refractory to depletion. Horikawa et al . [65] have demonstrated that B-cell depletion in lymphoma left endogenous IL-10-producing B cells, which impaired therapeutic efficacy. This suggests that Breg cells have a means to resist depletion by αCD20 therapy, similar to PD-L1 hi B cells. Adoptive transfer experiments of RTX-refractory PD-L1 hi B cells demonstrated suppressive activity, suggesting a novel mechanism by which RTX acts in disease. The refractory nature of PD-L1 hi B cells to RTX suggested that these cells retained a strong anti-apoptotic phenotype. Recent evidence suggests that post-RTX treatment, mice and patients have elevated levels of the B-cell survival factor, BAFF. This survival factor is known to drive Bcl2 and Bcl-XL, both anti-apoptotic factors which enhance cell survival [66] . Previous studies have indicated that suppression of Bcl2 increases the sensitivity of B cells to RTX treatment [67] . PD-L1 hi B cells exhibited high expression of the BAFF receptors BAFF-R, TACI and BCMA, with increased sequestration of BAFF. Blockade of BAFF-R led to elimination of PD-L1 hi B cells that is indicative of the increased efficacy seen with αCD20/BAFF-R co-treatment [55] , and that PD-L1 hi B-cell survival is BAFF dependent. Beyond their ability to directly suppress antibody responses and the evidence of their broad suppressive capacity, future investigations are required to decipher whether PD-L1 hi B cells have a key role in B-cell fate decisions. For example, PD-L1 hi B cells may direct the differentiation of GC B cells away from plasma cells into memory B cells, which would be suggestive of a role in vaccine efficacy. PD-L1 hi B-cell resistance to B-cell depletion therapy, a mainstay of the autoimmune therapeutic stratagem, demonstrates a unique mechanism of action that could have broad implications in many autoimmune diseases. In addition, analyzing the number of PD-L1 hi B cells may be used to predict the quality and quantity of humoral immune responses in vivo . A recent study by Cubas et al . [7] , found a higher frequency of PD-L1 + B cells in the GCs of lymph nodes from HIV-infected individuals, suggesting a potential role for PD-1–PD-L1 interaction in regulating T FH -cell function. It is highly plausible that elevated PD-L1 hi B cells are involved in this effect. Furthermore, therapy with PD-L1 hi B cells has potential for patients suffering from autoimmunity. Ex vivo data described above indicates the presence of these cells in man, demonstrating their homoeostatic existence. As seen in murine models, PD-L1 hi B cells are refractory to RTX therapy and have a suppressive role on peripheral T-cell activation. In summary, high PD-L1 expression on B cells defines a mechanism for potent suppression of humoral immunity through the regulation of T FH cells. Further work is needed to determine their ontogeny, relationship to previously defined Breg cells and how these cells may be used therapeutically to enhance protective immunity and long-term memory or to inhibit autoimmune diseases. Mice C57BL/6 strain mice were used in all studies. μMT −/− , Il10 −/− , Rag1 −/− , 2D2 (TCR MOG ), OT-II (TCR OVA ), Ptprc a (CD45.1 + ) and Prdm1 (Blimp1) – eYFP transgenic mice, all belonging to the C57BL/6 strain background, were from the Jackson Laboratory (Bar Harbor, ME, USA) and bred in-house. Pdl1 −/− (ref. 68 ), 10BiT mice [28] and DEREG mice [32] , all belonging to C57BL/6 strain background, were also bred in-house. All mice were bred in a specific pathogen-free barrier facility with female mice used at 6–10 weeks of age. All animal experiments were performed in compliance with the Irish Medicine Board regulations and approved by the Trinity College Bioresources Ethical Review Board. Human peripheral blood Peripheral blood from consenting healthy volunteers (aged 24–34 yrs old) was drawn and placed into heparinized vials (Vacuette). For BAFF uptake studies, B cells were isolated from peripheral blood via Histopaque-1077 (Sigma) density centrifugation and CD19 + magnetic selection (Miltenyi Biotec). Blood was obtained under ethical approval by the Trinity College Faculty Research Ethics Committee. Immunization Mice were immunized subcutaneously in a rear footpad with OVA adsorbed onto Alum (25 μg per site) or the tail base (100 μl each mouse) with 0.25 mg ml −1 KLH (Calbiochem) or 1 mg ml −1 MOG 35–55 emulsified in CFA (Sigma-Aldrich), as described previously [16] . Mice were killed on Day 14 following immunization. Experimental autoimmune encephalitis EAE was induced as described previously [69] . Briefly, mice were immunized subcutaneously with 200 μl of mixed 1 mg ml −1 MOG 35–55 /CFA with 2 mg ml −1 of heat-killed mycobacterium tuberculosis H37Ra (Hooke Laboratories). Mice were then challenged with intraperitoneal injection of pertussis toxin (Hooke Laboratories) 2 and 26 h after immunization. Clinical signs of EAE were assessed as follows: 0, no signs; 1, flaccid tail; 2, impaired gait/righting reflex; 3, hind limb paralysis; 4, total limb paralysis and 5, moribund or dead. For Ig assessment, mice underwent submandibular bleeding once a week. Animals showing a 20% body weight loss and/or sustained front leg impairment were humanely removed from the study in accordance with ethical regulations. The study was ended at D+26 as the humane end point of the experiment was reached. To isolate tissue for histology, mice were perfused through the left cardiac ventricle with 20 ml of cold PBS before spinal cords were flushed out by hydrostatic pressure using a syringe attached to a 19-gauge needle. Spinal cords were placed in 4% paraformaldehyde. Tissues were processed and blocked in paraffin wax. Transverse sections of the spinal cord were stained with Luxol-Fast Blue and eosin. Areas of demyelination were assessed for Luxol-Fast Blue-stained sections. Images were acquired using the Aperio scanscope. For CNS cell isolation, spinal cords were flushed out by hydrostatic pressure using a syringe attached to a 19-gauge needle. CNS tissue was then cut into small pieces and digested with collagenase A (2 mg ml −1 , Roche Diagnostics) and DNase (1 mg ml −1 , Sigma-Aldrich) at 37 °C for 45 min. Mononuclear cells were isolated by passing the tissue through a cell strainer (70 μm). Mononuclear cells were then counted to enumerate CNS cell infiltration by an investigator blinded to the experimental groups using Trypan Blue. To measure antigen recall responses at D+14 and D+26, single-cell suspensions of dLNs were cultured in the presence of RPMI-1640 (Invitrogen) supplemented with 10% heat-inactivated FCS (Sigma-Aldrich), 2 mM L-glutamine (Invitrogen), 50 IU ml −1 penicillin, 50 μg ml −1 streptomycin (Invitrogen), 10 mM HEPES (Sigma-Aldrich), 0.1 mM non-essential amino acids (Sigma-Aldrich), 50 μM 2-mercaptoethanol (Sigma-Aldrich) and 10 μg ml −1 MOG 35–55 peptide for 72 h. Mixed-bone marrow chimera generation Mice with a B-cell-specific PD-L1 deficiency were generated using the mixed-bone marrow chimera system. In brief, irradiated μMT mice (dose of 9 Gy (in two divided doses, 3 h apart) were reconstituted with a mixed inoculum of bone marrow (20% Pdl1 −/− or WT and 80% μMT; 1 × 10 7 cells transferred). The haematopoietic compartment was left for 8–10 weeks to repopulate. Thus, all B cells arising from these inocula originated from the Pdl1 −/− (or WT) portion, with all other haematopoietic lineages deriving predominantly from the μMT portion (that is, PD-L1 sufficient). These mice were designated B-PD-L1 −/− and B-WT chimeras. Chimerism was confirmed by flow cytometry, using CD3-FITC (17A2), CD19-PE-Cy7 (1D3) and PD-L1-APC (10F.9G2) antibodies. Characterization of chimeras is outlined in Supplementary Fig. 1 . Adoptive transfer experiments PD-L1 B-cell subsets were isolated by cell sorting, see below, and were transferred at three different cell doses (1 × 10 5 , 5 × 10 5 , 1 × 10 6 ) into WT, Pdl1 −/− or DEREG mice. For EAE studies, 1 × 10 6 PD-L1 hi B cells were transferred either D−7 or D+7 immunization. For T REG depletion studies, CD4 + FoxP3 + T cells were depleted from DEREG mice [32] by intraperitoneal injection of 1 μg DT 18 h before immunization with subsequent treatment 7 days post KLH/CFA administration. For transfers into μMT −/− mice, a total of 1 × 10 7 B cells were transferred. Animals were grouped into those that received no PD-L1 hi B cells, those that received a mixture that contained 5.2% PD-L1 hi B cells (as per homoeostatic conditions described above) and those that received a mixture that contained 25% PD-L1 hi B cells. For cell transfers in Rag1 −/− animals, 4 × 10 6 CD4 + T cells from TCR MOG or TCR OVA mice, and 4 × 10 6 B-cell subsets from either WT or Pdl1 −/− mice were used. In all cases, cells were injected intravenously and mice were left to reconstitute for 4 weeks prior to immunization with the appropriate antigen. For tracking studies, PD-L1-expressing B-cell subsets were isolated from the spleen of CD45.1 + transgenic mice and transferred via either the intravenous or intraperitoneal route into CD45.2 + mice. Flow cytometry—murine cells Single-cell suspensions from spleen and inguinal lymph nodes (dLN) were prepared and surface marker expression on cells was assessed by flow cytometry or used for cell sorting as described. Cells were washed in flow cytometry staining buffer (PBS with 2% FCS and 0.02% sodium azide) followed by blocking with anti-mouse CD16/32; used at a 1/1,000 dilution, 10 μl per sample (clone 93; eBioscience). For staining of blood, mAbs were added to whole blood before 20 min of lysis using Pharmlyse (BD Biosciences). The following mAbs are from BD Biosciences, CD3-FITC (17A2), CD5-BV510 (53-7.3) CD19-APC/PE-Cy7/V450 (1D3), CD21-FITC (7G6), CD95-biotin/PE-Cy7 (Jo2), CD138-PE (281-2), CXCR5-PE-Cy7 (2G8), PD-1-BV421 (J43), B220-APC-Cy7 (RA3–6B2) and IgD-PE (11–26c.2a); eBioscience: CD4-FITC (RM4–5), CD23-PerCP-eFluor710, ICOS-PE-Cy5 (7E.17G9), IL-21R-PE (eBio4A9), IgM-APC-eFluor780 (II/41) and GL-7-eFluor450 (GL-7); Biolegend: PD-L1-biotin/PE/APC (10F.9G2); Miltenyi Biotec: CD19-VioBlue (6D5), CD267-PE (8F10) and CD268-FITC (7H22-E16); R&D systems: BCMA/TNFRSF17-Fluorescein (161616) were used at a dilution of 1/100, 10 μl per sample . Streptavidin-PE, Streptavidin-PE-CF594 or Streptavidin-APC (BD Biosciences) was used as a secondary antibody for biotin labelling at a dilution of 1/200, 10 μl per sample . For transcription factor staining, cells were fixed and permeabilized with a commercial transcription factor staining kit (eBioscience) according to the manufacturer’s instructions, and the cells were stained with the following transcription factors (dilutions are specified in brackets, 10 μl per sample) from BD Bioscience—T-bet-AlexaFluor647 (O4–46; 1/200), Foxp3-PE (MF23; 1/100) Rorγt-BV421 (Q31–378; 1/100) and from eBioscience—Bcl-6-PE-CF594 (K112-91; 1/100) and Gata3-PE (TWAJ; 1/100). For detection of intracellular IL-21, cells were fixed and permeabilized with a commercial intracellular cytokine detection kit (BD Biosciences) according to the manufacturer’s instructions, and stained with IL-21-eFluor660 (FFA21; 1/200, 10 μl per sample; eBioscience). Viable cells were distinguished using LIVE DEAD Aqua (Life Technologies) at a dilution of 1/1,000, 20 μl per sample . Populations of interest were gated according to appropriate ‘fluorescence minus one’ controls. Samples were acquired on a CyAn flow cytometer (Beckman Coulter, CA, USA) and were analyzed with FlowJo software (Tree Star). Flow cytometry—human cells Heparinized whole blood was stained with the following antibodies. The following mAbs are from BD Biosciences: CD19-FITC (HIB19), CD27-PE-CF594 (M-T271), PD-1-BV421 (MIH18) and PD-L1-PE-Cy7 (MIH1), eBioscience: CD10-APC (SN5c), CD21-FITC (HB5), CXCR5-PE (MU5UBEE), ICOS-APC (ISA-3); Miltenyi Biotec: CD4-PerCP (VIT4), CD19-APC-Vio770 (LT19), CD267-PE (1A1), CD268-FITC (11C1) were used at a 1/10 dilution, 10 μl per sample. Following staining, blood was lysed using PharmLyse (BD Biosciences). Viable cells were distinguished using LIVE DEAD Aqua used at a 1/1,000 dilution, 20 μl per sample . For transcription factor staining, cells were fixed and permeabilized with a commercial transcription factor staining kit (eBioscience) according to the manufacturer’s instructions, and the cells were stained with BCL-6-PE-CF594 (K112-91; 1/10 dilution, 10 μl per sample, BD Biosciences). Populations of interest were gated as above. Samples were acquired on a CyAn flow cytometer and were analyzed with FlowJo software. Cell sorting For adoptive cell transfer experiments, spleen cells from mice were stained with PD-L1-PE, CD3-FITC and CD19-APC for B-cell sorting, and CD3-FITC, CD4-PE for T-cell sorting, on a MoFlo cell sorter (Beckman Coulter). Antibodies were used at the dilutions described above. Whole B cells were gated as CD3 − CD19 + before discrimination of PD-L1-expressing populations. For phenotypic analysis, spleen cells from KLH/CFA-immunized Prdm1– eYFP mice were stained for PD-L1-APC, CD19-V450, CD138-PE and B220-APC-Cy7 at dilutions described above. Live cells were distinguished and gated via Propidium Iodide (Sigma) staining (used at a 1/1,000 dilution). Routinely the purity of sorted cell populations was >97%. Sorted cells were used for adoptive transfer experiments or in vitro cell culture. Ex vivo human blood assay For T FH assays, heparinized whole blood was stimulated with 1 μg ml −1 SEB for 3 days. For ex vivo B-cell depletion studies, whole blood was cultured for a maximum of 5 days. Serum was taken for cytokine and Ig analysis at respective time points. mAb treatment For murine B-cell depletion studies, a single 250 μg murine αCD20 (I8BI2, Biogen Idec), was injected intravenously with IgG2a used as an appropriate ISO control. To determine the role of BAFF, 250 μg αBAFF-R (9B9, Adipogen) was also administered intravenously 8 days post αCD20 therapy. For in vitro blocking mAb cell-culture assays, cells were treated (0, 0.01, 0.1, 1 and 10 μg ml −1 ) with αPD-L1 (MIH5), αPD-L2 (TY25) and αPD-1 (J43; eBioscience). For human ex vivo B-cell depletion, RTX (αCD20 mAb, Genentech) was added to whole blood at either 1or 10 μg ml −1 as described. Mouse IgG1 was used as an appropriate ISO control. Human αPD-L1 (29E.2A3, Biolegend) was used at 1 or 10 μg ml −1 . Detection of phosphorylated proteins Co-cultures of CD4 + T cells and CD19 + B cells were stimulated using 1 μg ml −1 SEB (Sigma) for 5 days in cell-culture media. Post-stimulation cultures were re-activated with 40 nM phorbol 12-myristate 13-acetate for 15 min and fixed using BD-Phosflow Fix Buffer (BD Biosciences) at 37 °C. After washing in flow cytometry staining buffer, cells were permeabilized with BD-Phosflow Perm Buffer III (BD Biosciences) for 30 min before being stained with one of the following antibodies from BD Biosciences (used at a 1/50 dilution, 20 μl per sample); Akt(pS473)-AlexaFluor647 (M89-61), Stat3(pY705)-AlexaFluor647 (4/P-STAT3) or Stat5(pY694)-AlexaFluor647 (47/Stat5(pY694)). Populations of interest were gated as above. Samples were acquired on a CyAn flow cytometer and were analyzed with FlowJo software. BAFF uptake To determine BAFF uptake in both mouse and human B cells, recombinant BAFF (R&D Systems) was labelled with the AlexaFluor647 (AF647) microscale protein labeling kit (Life Technologies) as per manufacturer’s instructions. BAFF protein concentration, post labelling, was evaluated using a Nanodrop Spectrophotometer and compared against a standard curve of bovine serum albumin (Sigma). Isolated B cells, as described above, were treated with labelled BAFF at 0, 0.1, 1, 10, 100 and 1,000 ng ml −1 . Cells were analyzed via flow cytometry at time points (0, 1,3 and 5 h) for AlexaFluor647-associated cells as calculated by the median fluorescent intensity of AF647. Cytospins Isolated cells were spun onto poly-lysine-coated slides at 850 g for 2 min. Histological staining of cytospin samples was conducted using the Kwik-Diff stain kit (Thermo Scientific) as per manufacturer’s instructions. Images were acquired using a × 63 objective on a Leica DM3000 microscope. PD-L1 B-cell subset characterization Spleens from WT mice were collected and single-cell suspensions were created as described above. B cells were using the B220 microbead kit via AutoMACS (Miltenyi Biotec). Purity was determined by flow cytometry at 95%. Isolated cells were characterized via flow cytometry as described above. For cytokine profiles, B cells were cultured at a concentration of 2 × 10 6 cells per ml in culture media as described above. Cultures were stimulated with 5 ng ml −1 phorbol 12-myristate 13-acetate and 50 ng ml −1 ionomycin (Sigma-Aldrich) for 18 h. Supernatants were collected for analysis. For cell proliferation assays, B cells were isolated as described above and stained with Cell Proliferation Dye eFluor450 (eBioscience) at a final concentration of 5 μM as per manufacturer’s instructions. Cells were stimulated with either 20 μg ml −1 lipopolysaccharide (Sigma-Aldrich), 5 μg ml −1 ODN 1826 CpG (Invivogen) or 10 μg ml −1 αCD40 with 10 μg ml −1 αIgM (BD Biosciences). The degree of cell proliferation was assessed 5 days post stimulation via flow cytometry. Murine antibody detection Total IgG (cell-culture supernatants) and KLH-specific/MOG 35–55 -specific (serum) IgG, IgG1, IgG2a were determined by enzyme-linked immunosorbent assay (ELISA). In brief, high-binding 96-well microplates (Greiner Bio-One, Germany) were coated overnight at 4 °C with 2 μg KLH or 5 μg MOG 35–55 per well or the appropriate anti-mouse capture Ab (BD Biosciences), blocked with 1% bovine serum albumin/PBST, and incubated with appropriate dilutions of sera or culture supernatant. Bound Ig was detected using the appropriate biotin-conjugated rat anti-mouse Ig (BD Biosciences) followed by streptavidin–horseradish peroxidase conjugate (R&D Systems) and o -phenylenediamine dihydrochloride (Sigma-Aldrich) substrate. Absorbance at wavelength 490 nm was read using a microplate reader (VersaMax tunable microplate reader; Molecular Devices, Sunnyvale, CA, USA). Human IgG detection Total serum IgG was determined via ELISA using the Total IgG Ready-SET-Go kit (eBioscience) as per manufacturer’s instructions. For all IgG quantification, dashed lines, where visible, represent the detection limit. Murine cytokine detection IL-2, IL-4, IL-6, IL-10, IL-12p70, IL-17, IFN-γ and CXCL13 from cell-culture supernatants and serum BAFF levels were determined via ELISA (R&D Systems) as per manufacturer’s instructions and described above. For all cytokine data, dashed lines, where visible, represent the detection limit. Human cytokine detection Serum IL-6, IL-21 (Ready-SET-Go) and BAFF were determined via ELISA as per manufacturer’s instructions and described above. For all cytokine data, dashed lines, where visible, represent the detection limit. Statistical analysis Experiments were adequately powered using the law of diminishing return with sample sizes based on previous studies. Subjects were randomly selected for participation in experimental groups. All data are shown as mean±s.e.m. Variances were calculated prior to statistical comparison. Specific statistical tests are described in figure legends. How to cite this article: Khan, A. R. et al . PD-L1 hi B cells are critical regulators of humoral immunity. Nat. Commun. 6:5997 doi: 10.1038/ncomms6997 (2015).